A signal peptide peptidase is required for ER-symbiosome proximal association and protein secretion During legume-rhizobia symbiosis, differentiation of the symbiosome (engulfed intracellular rhizobia) is necessary for successful nitrogen fixation. To control symbiosome differentiation, host cell subcellular components, e.g., ER (endoplasmic reticulum), must adapt robustly to ensure large-scale host protein secretion to the new organelle. However, the key components controlling the adaption of ER in nodule cells remain elusive. We report that Medicago BID1 , a nodule-specific signal peptide peptidase (SPP), is central to ER structural dynamics and host protein secretion. In bid1 , symbiosome differentiation is blocked. BID1 localizes specifically to the ER membrane and expresses exclusively in nodule cells with symbiosomes. In the wild type ER forms proximal association structures with symbiosomes, but not in bid1 . Consequently, in bid1 excessive ER stress responses are induced and ER-to-symbiosome protein secretion is impaired. In summary, a nodule-specific SPP is necessary for ER-symbiosome proximal association, host protein secretion, and symbiosome differentiation. The nitrogen-fixing symbiosis (NFS) between legumes and rhizobia ensures plants an efficient way to get fixed nitrogen. During NFS, plants form a specific organ, the root nodule, to host their microbial partners. Inside nodules, rhizobia fully enter host cells, are encapsulated by a plant-derived lipid membrane, and form a subcellular organelle-like structure, the symbiosome (rhizobia within symbiosome is termed bacteroid) [1] . Once fully settled inside host cells, symbiosomes surrender the control of their fate to hosts, to a great degree. In Inverted Repeat-Lacking Clade (featured by the loss of a 25-kilobase inverted repeat in the chloroplast genome) species such as the model legume Medicago truncatula , symbiosomes undergo terminal differentiation, which is characterized by drastic changes in genome ploidy, morphology, transcriptional, metabolic patterns and lost abilities of propagation [2] . As a prerequisite for successful NFS (free-living rhizobia and undifferentiated symbiosome cannot fix nitrogen), symbiosome differentiation is initiated and regulated by host secreted proteins [2] , [3] . Large numbers of host-secreted proteins have been identified. In Medicago, host cells secrete NCR ( N odule-specific C ysteine R ich) peptides, nodule-specific GRP ( G lycine R ich P eptides), and many others [4] , [5] , [6] , [7] , [8] , to promote symbiosome differentiation. High-throughput trafficking of host proteins is controlled by a nodule-specific protein secretory pathway [3] . Through alternative cleavage and polyadenylation, host cells generate a nodule-specific isoform of SYP132 (SYNTAXIN 132), which marks the symbiosome membrane, the interface between host cell and bacteroid, to guide host protein trafficking [9] , [10] . Several key regulators of host-to-symbiosome vesicle trafficking have also been reported [11] , [12] . Considering the importance of symbiosome differentiation to this symbiosis, research into nodule cell-specific protein secretion is critical to our understanding of the NFS. ER (endoplasmic reticulum) is a sub-cellular organelle central to intracellular protein production and secretion. Its structure is highly dynamic, moreover, the ER forms direct membrane-to-membrane structures for interaction with other organelles, including mitochondria, Golgi, and the plasma membrane, to transport lipids and other molecules [13] , [14] . During NFS, the ER plays a key role in accommodating and communicating with symbiosomes, with the aforementioned host protein secretion as the most prominent example. While symbiosome-destined host proteins are diverse in their sequences and structures, most of them have a N-terminal signal peptide (SP) in their nascent sequences, which is cleaved by the DNF1 nodule-specific Signal Peptidase Complex (SPC) at the ER membrane, to facilitate proper folding and secretion [6] , [15] . More than controlling protein production and secretion, early studies suggest that ER tubes are spatially close to membranes of differentiated symbiosomes [16] , and there are reports of ER structural adjustments in rhizobial infection and symbiosome development [17] , [18] , [19] . The mechanism beneath robust ER adaption to assert the delicate control of host protein secretion and host-symbiosome communication remains elusive. A more specific question is related to SPs, upon SP excision, it remains unknown how nodule cells cope with SP fragments on ER membrane, to ensure proper ER function and protein secretion. Here we report that in nodule cells, a nodule-specific signal peptide peptidase (SPP) at the ER membrane is necessary for proper ER structural reconfiguration, successful host protein secretion, and NFS. Symbiosome differentiation is blocked in bid1 To find key genes regulating symbiosome differentiation, we screened for mutants with a “ bacteroids with impaired differentiation ” phenotype ( bid mutants). Medicago truncatula line NF-FN6798 (named bid1 here), a fast neutron bombardment mutant from the Noble Research Institute, the United States, had white, round and small nodules (Fig. 1a , Supplementary Fig. 1a ). In bid1 , nodule cells were smaller, symbiosomes were undifferentiated and less orderly arrayed (Fig. 1b , Supplementary Fig. 1b , c ). Confocal microscopy and TEM assays confirmed that in bid1 cells, rhizobia within symbiosomes failed to differentiate (Fig. 1 c, d , Supplementary Fig. 1d ), reminiscent of dnf1 defects [15] . Furthermore, in the analysis of isolated symbiosomes, indeed bid1 symbiosomes were smaller and less elongated (Fig. 1e ), their length in bid1 was much lower compared to WT (Fig. 1g ). Consistent with defects in differentiation, in bid1 the expression levels of NCR001 and NCR169 , two representatives of differentiation-promoting NCR peptides, were much lower (Fig. 1h , Supplementary Fig. 1e ). Moreover, expression levels of several key rhizobial genes were altered in bid1 nodules. exoY encodes an enzyme required in early steps of exopolysaccharide synthesis [20] ; ctrA is a key transcription factor controlling bacterial cell cycle [21] ; and bacA encodes a membrane protein protecting rhizobia from antimicrobial molecules, e.g., NCR peptides [22] . The expression levels of exoY , exoB , ctrA and bacA were much higher compared with WT (Fig. 1 i, j , Supplementary Fig. 1 f, g ), indicating altered states of exopolysaccharides synthesis and impaired differentiation of bacteroids in bid1 cells [23] , [24] , [25] . Consequently, rhizobial nifH::GUS reporter was not activated in bid1 nodules (Fig. 1f ). These results show that in bid1 , symbiosome differentiation is blocked at an early stage upon symbiosome formation. Fig. 1: Symbiosome differentiation is impaired in nodule cells of bid1 . a bid1 mutant only had small and white nodules when inoculated with S. meliloti ABS7 hemA::LacZ . Representative pictures of nodules were taken at 21 dpi (days post inoculation). Bar=1 mm. b Symbiosomes were not differentiated in bid1 nodule cells from a in nodule sectioning assay. Note that infected bid1 nodule cells were also smaller than WT. Nodules from a were sectioned into 5 μm slides and stained with toluidine blue. Bar=20 μm. c Symbiosomes in bid1 nodule cells were undifferentiated. 21 dpi nodules inoculated with S. meliloti RM021 pHC60-GFP were stained with PI (Propidium iodide, red) and analyzed under confocal microscopy. Bar=10 μm. d Symbiosomes were undifferentiated in bid1 nodule cells in TEM assay. 21 dpi nodules inoculated with ABS7 hemA::LacZ were used for analysis. Letter “b” indicated bacteroids. Bar=2 μm. e Representative pictures showing differences between isolated symbiosomes from WT and bid1 . Symbiosomes were isolated from nodules in c . Bar=10 μm. f bid1 symbiosomes were much shorter in length in the quantification assay of symbiosomes from e . Piano plot to show the minimum, 25th percentile, median, 75th percentile and maximum symbiosome lengths. Numbers of symbiosome analyzed were indicated respectively. “***”, P < 0.0001 in one-way ANOVA assay. g nifH::GUS reporter was not activated in bid1 nodule cells. GUS staining was performed on WT and bid1 nodules 21 days after inoculation with S. meliloti RM1021 nifH::GUS at 21 dpi. Bar=750 μm. h , Expression of NCR001 was totally blocked in bid1 nodule cells. qRT-PCR assay was performed using samples from nodules 21 dpi with ABS7 hemA::LacZ . ND, not detected. i and j, Rhizobium ExoY and CtrA genes were highly expressed in bid1 nodule cells compared with WT. qRT-PCR assays were done using the same samples as in h . For h, i and j , “**” and “***” meant P < 0.01 and P < 0.001 in Student’s t -test, respectively. Data were represented as means ± SEM of three independent amplifications. Experiments were repeated at least 3 times with similar results. Full size image BID1 encodes a nodule-specific SPP To identify the BID1 gene, we performed a bulked segregation assay using the F2 population of bid1 crossed to WT A20. bid1 mutation was mapped to the upper arm of Chromosome 1, close to marker 001e11 (Fig. 2a ). Subsequently We performed whole genome sequencing of bid1 . In bid1 , a 8857 bp fragment from Chromosome 2, 44,572,921 to 44,581,777 bp, is translocated onto Chromosome 1, next to the adenine at 877,946 bp (Fig. 2a ). The translocation is within the 5’ UTR region of MtrunA17_Chr1g0147151 (Medtr1g008280 in Mt4.0), at 102 bp upstream of the start codon (Fig. 2a ). The expression of target gene was significantly reduced (Supplementary Fig. 1h ), proving translocation-caused transcriptional inactivation. Expressing the genomic sequence of the target gene with a N-terminal GFP tag in bid1 could complement the “fix-” phenotype (Fig. 2b ), confirming bid1 phenotype is caused by the defect in MtrunA17_Chr1g0147151 gene. Fig. 2: BID1 encodes a nodule-specific, ER membrane-localized SPP. a A diagram showing BID1 gene structure and the position of the target mutation in rough mapping. BID1 was mapped to the upper arm of Chromosome 1, in the interval between markers 001e_01 and h2_116k17a. A 8,857-bp fragment from Chromosome 2, 44,572,929-44,581,777 bp, is inserted into the 5’ UTR of MtrunA17_Chr1g0147151 , 102 bp ahead of the start codon. b Expressing GFP -fused candidate gene genomic sequence driven by its own promoter could complement the bid1 phenotype. Please note that GFP tag need be inserted at N-terminus of BID1. Bar=2 mm. c BID1 is a multi-transmembrane domain-containing SPP protein. The transmembrane domains were shown, and two conserved aspartate residues critical for peptidase activity were labeled red. PAL, a conserved motif important for peptidase activity; KKXX, the C-terminal ER membrane localization signal. Numbers indicated positions of the amino acids. d BID1 is expressed exclusively in nodules in promoter-GUS reporter assay. Zone I, nodule meristem, Zone II, infection zone, the zone rhizobia infect nodule cells, Zone III, differentiation zone, the zone where symbiosomes undergo differentiation, Zone IV, fixation zone, the zone symbiosomes fix nitrogen. Bar=500 μm. e BID1 localized specifically at ER membrane when expressed in the leaves of Nicotiana benthamiana . N. benthamiana leaves co-transformed with 35 S::GFP-BID1 and mCherry-HDEL ER reporter were analyzed under confocal microscopy at 2 days post-transformation. Bar=10 μm. f , BID1 localized to the ER membrane in nodule cells. A construct expressing pBID1::GFP-BID1 together with mCherry-HDEL reporter was transformed into bid1 mutants. Bar=10 μm. g and h Fluorescent intensity measurement of GFP-BID1 and mCherry-HDEL in indicated regions of tobacco leaf and nodule cells respectively. Fluorescent peaks of GFP-BID1 overlapped with mCherry-HDEL signals in both cell types. Fluorescent intensity was measured as grey value of pixels using ImageJ software. Roi, region of interest. Experiments were repeated more than 3 times with similar results. Full size image BID1 is annotated to encode a SPP, an aspartic endopeptidase with intra-membrane protein cleavage activity [26] , [27] . As a critical component for ER protein secretion, SPP digests remnant SPs inside the ER membrane upon SPC-mediated release of SPs from nascent polypeptides [28] , [29] . BID1 protein contains 8 transmembrane domains, with two conserved aspartate residues in the middle of the 5th and 6th transmembrane, respectively (Fig. 2c ) [29] . The C-terminus of BID1 contains a conserved KKXX motif, which is critical for ER-membrane localization of many ER resident proteins (Fig. 2c ) [30] . By searching the Alphafold2 protein structure database [31] , we found the predicted BID1 structure was identical to that of human SPP protein (Supplementary Fig. 1i ), further confirming BID1 functions as a SPP. Key genes regulating symbiosome differentiation are usually nodule-specifically expressed [32] . A β-glucuronidase (GUS) reporter assay was performed to investigate the expression pattern of BID1 . pBID1::GUS activity was detectable only in nodules, in every nodule zone except meristem, indicating BID1 is a nodule-specific gene (Fig. 2d ), which was also confirmed by analyzing public RNA-Seq and Microarray data (Supplementary Fig. 2a , b ). Moreover, BID1 is expressed in close correlation with DNF1 , a representative of nodule-specific SPC (Supplementary Fig. 2a-c ) [15] , similar cis elements were identified in promoter regions of BID1 and DNF1 (Supplementary Fig. 2d , 2e ). The expression pattern of BID1 is consistent with its fundamental roles in symbiosome differentiation, also transcriptionally it may be activated together with DNF1 . BID1 is a multi-pass membrane protein. We expressed GFP-BID1 fusion sequence driven by 35 S promoter together with mCherry-HDEL , the widely used ER marker [33] , in Nicotiana benthamiana leaves. GFP-BID1 had an ER web-like distribution pattern and co-localized with mCherry-HDEL (Fig. 2e, g ), showing BID1 probably localizes at ER membrane. To confirm BID1 localization in nodule cells, we transformed bid1 with a construct expressing GFP-BID1 fusion sequence under BID1 promoter and Arabidopsis UBQ10 -driven mCherry-HDEL reporter together. This construct could also complement bid1 phenotype (Supplementary Fig. 2f ). Under confocal microscopy, GFP-BID1 co-localized well with mCherry-HDEL (Fig. 2f, h ), proving BID1 is an ER membrane protein in nodule cells. When GFP was fused to BID1 at the C-terminus, BID1-GFP could not complement bid1 (Fig. 2b ). The KKXX motif is required strictly at the C-terminus for successful ER membrane localization [30] , fusing GFP to the C-terminus would have blocked proper BID1 targeting. In GFP-BID1 nodules, GFP signals could only be detected in large cells (Supplementary Fig. 2g ). As symbiosome-containing cells tend to be larger, BID1 may only exist in cells infected by rhizobia. When GFP-BID1 plants were inoculated with Rm1021 mCherry strain, indeed GFP-BID1 was specifically restricted to cells containing symbiosomes (Supplementary Fig. 2h ), proving BID1 expresses exclusively in infected cells. BID1 evolves from a housekeeping homolog Key to the ER protein secretory apparatus, SPP is highly conserved among yeast, mammalians and plants [29] . As BID1 only expressed in nodules (Fig. 2d ), we searched for its housekeeping homologs. In Medicago, BID1 has one homolog with a highly similar sequence (Supplementary Fig. 3a ), which we named BID1-Like ( BID1L ). The gene structure of BID1L is also highly similar to BID1 (Supplementary Fig. 3b ). Unlike BID1 , BID1L expression is similar across Medicago tissues (Supplementary Fig. 3c ). BID1 probably evolved as a nodule-specific SPP basing on BID1L . To confirm this notion, we constructed a phylogenetic tree of BID1 and BID1L paralogs from moncots, dicots, including multiple legumes [1] . While BID1L paralogs could be found in every species (some have more than one copy), BID1 paralogs were specific to IRLC-clade species (Supplementary Fig. 4 ). This is similar to nodule-specific DNF1 [15] , indicating in IRLC-clade legumes, genes function in secretory pathway evolved nodule-specific duplicates to promote terminal symbiosome differentiation. ER stress responses are induced in bid1 As a SPP, BID1 functions to cleave SP fragments on ER membrane. Missing BID1 will probably cause accumulation of SP fragments, leading to excessive ER stresses and disturbance of ER functions [34] , [35] , [36] . To determine ER stress responses in bid1 , we checked the expression levels of ER stress marker genes, which tend to have multiple orthologues in Medicago (Supplementary Fig. 5a ). Majority of ER stress marker genes were significantly activated in bid1 nodules (Fig. 3a-e , Supplementary Fig. 5b-g ). Orthologues of bZIP28 and bZIP60 , two basic leucine zipper (bZIP) transcription factors [37] , [38] , [39] , were highly induced (Fig. 3a-c ). BiP3 ( bZIP induced protein 3 ) orthologues [40] , [41] , the ER-resident HSP70 cognates activated by bZIP28 and bZIP60 , were also highly expressed in bid1 (Figs. 3d, e ). Surprisingly the expression levels of BAG7c (homolog of Bcl-2-associated athanogene 7 ) [42] , and ERO1 ( Endoplasmic Reticulum Oxidoreductions 1 ) [43] , two genes necessary for proper maintenance of ER stress responses, were downregulated (Supplementary Fig. 5d , e ). We reason that in bid1 cells, ER stress responses are activated to some extent, in a unique way. How BID1 mutation leads to specific ER stress responses requires further investigation. Fig. 3: BID1 is required for proper ER-symbiosome proximal association. a-e In qRT-PCR assay a group of ER stress-related marker genes were induced in 21 dpi bid1 nodules inoculated with ABS7 hemA::LacZ . Error bars represent standard deviation from three biological replicates. “**” and “***”, P < 0.01 and P < 0.001 in Student’s t -test respectively. Data were represented as means ± SEM of three independent amplifications. f Confocal microscopy analysis of ER structures in WT and bid1 nodule cells. 14 dpi Rm1021 pHC60-GFP inoculated mCherry-HDEL-expressing WT and bid1 nodules were analyzed. For both panels, bar=10 μm. Roi, region of interest. g and h Fluorescent intensity of symbiosome GFP and ER mCherry signals of indicated regions in WT and bid1 respectively. Fluorescent intensity (grey value of pixels) was measured by ImageJ. i TEM assay results of ER and symbiosome structures in 14 dpi ABS7 hemA::LacZ- inoculated WT and bid1 nodule cells. For both panels, bar=1 μm. j Reconstructed 3D structures of symbiosomes and ER in WT and bid1 cells varied significantly. Overview of several ER and symbiosomes and zoomed-in structures of individual symbiosome and ER were shown. Symbiosomes were labelled in blue, ER in orange red. Structures were obtained through 3D reconstruction of AutoCUTS-SEM tomography data using Imaris software. Scal bar, 1 μm. k and l Piano charts showing differences in ER width and area between WT and bid1 , respectively. ER width and area in i were measured using ImageJ. “***”, P < 0.001 in One-way ANOVA assay. m Measurement of ER volumes in WT and bid1 by Imaris. “*”, P < 0.05 in one-way ANOVA assay. Numbers of ER analyzed were indicated. n Average distance between ER membrane and symbiosome was much larger in bid1 . ER-symbiosome distances were measured using Imaris. y-axis, logarithmic scores of ER-symbiosome distance to the base 2. “***”, P < 0.001 in one-way ANOVA assay. For k, l and n , numbers of ER analyzed were indicated. For m , 3D ER structures were evenly divided into 20 segments, volumes of each segment were determined. Experiments were repeated 3 times with similar results. Full size image ER-symbiosome proximal associations are impaired in bid1 cells ER is a large, membranous organelle functioning in protein and lipid production and secretion, its structure is highly dynamic and it can have distinct shapes [13] . To investigate disturbances to ER functions by undigested SP fragments and activated ER stress responses, we checked ER structures in WT and bid1 nodule cells. When stained by ER-Tracker Red, a chemical that stains ER membrane specifically, in infected WT cells, ER was highly expanded during cell development, and ER signals were in proximity with symbiosomes, a strong indication of ER structural remodelling during symbiosome differentiation (Supplementary Fig. 6 ). In bid1 , the ER was arranged irregularly throughout the nodules (Supplementary Fig. 6 ), indicating failed ER structural reconfiguration. We further determined ER structure using an mCherry-HDEL reporter. Overall ER structure varied significantly between WT and bid1 cells (Supplementary Fig. 7a ). In zone-by-zone comparisons, only in the infection zone were ER structural patterns similar between WT and bid1 (Supplementary Fig. 7b-h ). In WT differentiation and fixation zone cells, mCherry-HDEL labeled ER formed web-like structures, which expanded extensively and were in close proximity to GFP-labeled symbiosomes, while in bid1 , mCherry-HDEL signals were dot-like, and the ER failed to form regularly arrayed webs around symbiosomes (Fig. 3f-h , Supplementary Fig. 7b-h ). Neither WT nor bid1 uninfected cells form an extensive ER web in ER-tracker Red staining or ER fluorescent reporter assays, indicating cell type-specificity of ER structures (Supplementary Fig. 8a , b ). A TEM assay was performed to investigate the presumed ER-symbiosome association more thoroughly. Corroborating with confocal microscopy, in WT cells, there were a large number of ER sheets following symbiosomes closely (Fig. 3i ). In bid1 , relatively straight lines of ER were lost, ER structures were disordered and failed to associate closely with symbiosomes (Fig. 3i ), and ER width and area size were larger (Fig. 3 k, l ). Moreover we utilized serial AutoCUTS-SEM (Scanning Electronic Microscopy) and 3D topological reconstruction to build ER and symbiosome structural models. Notably in WT nodule cells, symbiosomes were completely encircled by dense ER lines (Fig. 3j , Supplementary Movie 1 , 3 ), with an average distance between the ER and symbiosome of several dozen nanometers (Fig. 3n ), well within the range of organelle membrane-membrane contact [13] , [14] . In bid1 cells, the ER was not structured as well-arrayed sheets and failed to surround symbiosomes (Fig. 3j , Supplementary Movie 2 , 4 ), the ER volume was much lower (Fig. 3m ), and average ER-symbiosome membrane distances were much larger (Fig. 3n ), indicating damaged ER structural construction and ER-symbiosome proximal association. Our results suggest that the ER of nitrogen-fixing nodule cells is closely associated with symbiosomes, and that this requires BID1. BID1 is required for host protein secretion The dissociation of ER and symbiosomes in bid1 suggests that host protein secretion may be impaired. To test this, we investigated ER-to-symbiosome secretion of several known host proteins. NCR001, a representative substrate of the DNF1 nodule-specific SPC [6] , NCR166, another NCR peptide expressed early during symbiosome differentiation (Supplementary Fig. 9a ), and CAML1 ( Calmodulin-Like 1 ), a member of the nodule specific calmodulin-like protein subfamily [5] , were expressed in WT and bid1 , respectively, under the BID1 promoter. BID1 promoter could activate the GUS reporter in bid1 mutant (Supplementary Fig. 9b ), indeed expression levels of NCR001-GFP , NCR166-GFP and CAML1-GFP transcripts were even higher in bid1 than WT (Supplementary Fig. 9c ). Confocal microscopy revealed that while in WT GFP-tagged NCR001, NCR166 and CAML1 localized to the symbiosome, likely the peri-bacteroid space, in bid1 these proteins could not be secreted (Fig. 4a , d, g). Similar results were obtained by analyzing individual symbiosomes (Fig. 4b, e, h ), further demonstrating blocked host protein secretion in bid1 . Confocal microscopy results were confirmed by Western blot analyses of isolated symbiosomes (Fig. 4c, f ), although we failed to detect CAML1-GFP. These results show that in bid1 mutant, host protein secretion is blocked, showing degrading SP fragments on the ER membrane is necessary for proper ER-to-symbiosome protein trafficking. Fig. 4: BID1 is required for the secretion pathway in nodule cells. a, d and g Secretion of NCR001, NCR166 and CAML1 were blocked in bid1 nodule cells. GFP -fused NCR001 , NCR166 and CAML1 were expressed under the BID1 promoter in WT and bid1 , respectively. 14-day-old nodules inoculated with S. meliloti Rm1021 mCherry were analyzed by confocal microscopy. Bar=10 μm. b, e and h GFP-fused NCR001, NCR166 and CAML1 could not be detected in bid1 symbiosome. Symbiosomes were isolated from nodules in a, c , and e respectively, and analyzed by confocal microscopy. Bar=5 μm. c and f , In Western blot assay of isolated symbiosome, secretion of NCR001 and NCR166 were blocked in bid1 nodule cells. GFP -fused NCR001 , NCR166 were expressed under BID1 promoter in WT and bid1 . Symbiosomes were isolated from 14-day-old nodules inoculated with ABS7 hemA::LacZ . Protein samples were subjected to Western blot. Protein amounts loaded in each sample were labeled. Experiments were repeated more than 3 times with similar results. Full size image In this work we report BID1, a nodule cell-specific SPP functioning at the ER membrane, is critical for symbiosome differentiation in nodule cells. Beyond illustrating SPP-mediated nodule-specific protein secretion (Fig. 4 ), the discovery of BID1 has broader impacts for our understanding of ER stress responses and ER-symbiosome proximal association during NFS (Fig. 5 ). Fig. 5: Diagram to summarize the function of BID1 in nodule cell ER reconfiguration and protein secretion. Nodule cells secrete a large number of proteins, e.g., NCR peptides, to symbiosomes to promote their differentiation. SP sequences could be found at the N terminus of these host proteins. The DNF1 nodule-specific SPC cleaves SP fragments from nascent sequences of host proteins to ensure proper folding and SYP132-mediated target protein secretion. On the ER membrane, remnant SP fragments will be cleaved by BID1, the nodule-specific SPP. In WT cells containing symbiosomes, ER forms an extensive web-like structure, closely surrounding differentiated symbiosomes. In bid1 mutant, with the nodule-specific SPP missed, ER structural reconfiguration and ER-symbiosomes proximal association are damaged, resulting in blockage of host protein secretion. In summary the nodule-specific SPP on ER membrane is critical for ER structural reconfiguration, ER-symbiosome proximal association, and host protein secretion. Full size image The Arabidopsis genome has one SPP, which is lethal if knocked out [34] . This is probably also be true for BID1L , the housekeeping SPP in Medicago, and SPP orthologues from other plant species. Thus bid1 holds unique and irreplaceable advantages in studying molecular links between mutations in SPP and ER stress responses, as in the mutant ER stress responses are activated in a unique way (Fig. 3a-e , Supplementary Fig. 5b-g ). ER structural adaption during symbiosome differentiation has been hinted long time ago [16] , [17] , [18] , [19] , yet the structural relationships between the ER and symbiosome are not clear. In maturing cells with symbiosomes, the ER forms an extensive web-like structure spreading throughout the cytoplasm (Fig. 3f-i ). Using AutoCUTs-SEM and 3D modelling, we show that the ER structure is closely associated with differentiating symbiosomes (Fig. 3j ), with the distance between ER and symbiosome well within the range of organelle contact (Fig. 3n ). In bid1 nodule cells, with the SPP missing, ER structure is significantly altered, the well-arrayed ER web, and in most cases, the ER-symbiosome proximal associations, are missing (Fig. 3i-n ), highlighting the impacts of BID1 on ER-symbiosome structural association. As exemplified by BID1 (Fig. 3f-n ), there might be a complete set of nodule-specific genes, which acquired their functions from their housekeeping homologs, that function in ER structural construction. The possible functions of ER-symbiosome proximal association are intriguing. The ER can form a close membrane-membrane interaction with every organelle and plasma membrane in various cell types, their direct interaction can facilitate trafficking of lipids and other molecules [13] , [14] . In infected cells of the fixation zone, mature symbiosomes occupy a large proportion of the cell volume (Figs. 1 c, d, 3f), ER-s ymbiosome proximal association may facilitate the transfer of lipids and other metabolites. For instance, since the bacteria are enveloped by a lipid membrane derived from plants [11] , certain lipids may be transferred to symbiosome through ER-symbiosome proximal association, as is the case of phosphotidylethanolamine transportation between ER and mitochondria in mammalian cells with the nutrients depleted [44] . Combining this work and earlier studies about ER adaption during NFS [16] , [17] , [19] , it is highly possible the ER and symbiosome form direct organelle contact structures in nodule cells (Fig. 3f-n ). To fully prove direct organelle contact between the ER and symbiosome, a tethering complex and its cargos should be identified. Nevertheless existence of the contact can be demonstrated, at least structurally, by findings of BID1-mediated ER-symbiosome proximal associations (Fig. 3f-n , Supplementary Fig. 7 ). Beyond signal peptide fragments, multiple substrates of human SPP have been reported [45] , [46] . It should not escape our attention that some cleaved products from BID1-mediated degradation of SP fragments may have novel functions in nodule cells, and BID1 may have a broader spectrum of substrates beyond SP, similar to scenarios in human cells [47] , [48] . Further investigations into BID1, particularly through the identification of its direct substrates by biochemical assays, will significantly contribute to fully revealing the molecular communications between nodule host cells and their microbial partner in the symbiosomes. Plant growth, rhizobia inoculation and hairy root transformation Medicago truncatula A17 and A20 plants were used in this study. Plants were grown in growth rooms at 22 °C, with 16 hours light (150 μE m −2 sec −1 ) and 8 hours dark. S. meliloti strains ABS7 hemA::LacZ , Rm1021 nifH::GUS , Rm1021 mCherry and Rm1021 pHC60-GFP were used for plant inoculation in this study. In brief, rhizobia collected from fresh overnight liquid culture were suspended in half basic nodulation medium (BNM), to the concentration of OD 600 = 0.05. 5 mL of liquid BNM culture were used for inoculation per plant in green zeolite. Agrobacterium rhizogenes strain Arqua1 was used for hairy root transformation of Medicago plants, the experiments were performed following previously described procedures [49] . To select transformed plant tissues, seedlings infected by agrobacteria strains were grown in Fahraeus medium containing 15 μg/mL kanamycin or 25 μg/mL hygromycin (antibiotics were chosen according to antibiotic resistance genes of the specific constructs) for 10 days. Map-based cloning, whole genome sequencing and complementation assays To map BID1 gene, bid1 mutant was crossed with WT A20 plants. F1 plants were inoculated with ABS7 hemA::LacZ to prove bid1 is a recessive mutation. In F2 population, seedlings were also inoculated with ABS7 hemA::LacZ . At 21 dpi, leaf samples from fix- and fix+ plants were collected respectively and subjected to bulked segregation analysis, using a group of genetic markers to determine the rough location of BID1 . Upon mapped BID1 to a unique locus on Chromosome 1, DNA samples were sent to BGI Shenzhen for whole genome sequencing using BGI sequencing platform. Whole genome sequencing data were analyzed using IGV software (Integrative Genome Viewer, https://software.broadinstitute.org/software/igv/ ). Two constructs were used to complement bid1 mutant with the target gene, pBID1::GFP-gBID1-pKGW-RR and pBID1::GFP-gBID1-UBQ10::mCherry-HDEL-pKGW . The constructs were transformed into bid1 mutants through hairy root transformation, transformed plants were inoculated with ABS7 hemA::LacZ and phenotypes were determined at 21 dpi. Molecular cloning In this study KOD Plus DNA polymerase (TOYOBO, Japan) was used to amplify target DNA fragments. The ligations were performed through In-fusion cloning using ClonExpress UltraOneStep Kit (Vazyme, China). For pBID1-pMDC163 construct, a 2.5 Kb fragment containing BID1 promoter and 5’ UTR was ligated into pMDC163 directly. To make the pBID1::GFP-gBID1-pKGW construct, GFP coding sequence was ligated into pUC18 vector, then the DNA fragment containing BID1 promoter and 5’ UTR and BID1 genomic sequence were ligated into GFP-pUC18 respectively. Then the pBID1::GFP-gBID1 sequence was amplified through PCR and ligated into pKGW . To make the pBID1::GFP-gBID1-UBQ10::mCherry-HDEL-pKGW construct, mCherry-HDEL was amplified and ligated with UBQ10 promoter, then the complete UBQ10::mCherry-HDEL sequence was amplified and ligated into pBID1::GFP-gBID1-pKGW . Meanwhile the UBQ10::mCherry-HDEL fragment was ligated into pKGW directly to generate the mCherry-HDEL reporter construct. For pBID1::gBID1-GFP construct, a DNA fragment covering BID1 promoter to the stop codon was amplified and ligated into pMDC107 , then the pBID1::gBID1-GFP fragment was amplified and ligated into pKGW . To express GFP -fused NCR001 , NCR166 and CAML1 in nodule cells, genomic sequences of the genes were amplified and ligated into pBID1-pKGW (a DNA fragment containing BID1 promoter and 5’ UTR sequence was ligated into pKGW in advance) respectively. 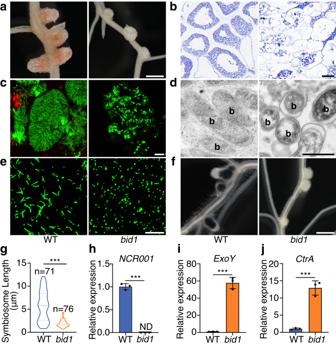Fig. 1: Symbiosome differentiation is impaired in nodule cells ofbid1. abid1mutant only had small and white nodules when inoculated withS. melilotiABS7hemA::LacZ. Representative pictures of nodules were taken at 21 dpi (days post inoculation). Bar=1 mm.bSymbiosomes were not differentiated inbid1nodule cells fromain nodule sectioning assay. Note that infectedbid1nodule cells were also smaller than WT. Nodules fromawere sectioned into 5 μm slides and stained with toluidine blue. Bar=20 μm.cSymbiosomes inbid1nodule cells were undifferentiated. 21 dpi nodules inoculated withS. melilotiRM021pHC60-GFPwere stained with PI (Propidium iodide, red) and analyzed under confocal microscopy. Bar=10 μm.dSymbiosomes were undifferentiated inbid1nodule cells in TEM assay. 21 dpi nodules inoculated with ABS7hemA::LacZwere used for analysis. Letter “b” indicated bacteroids. Bar=2 μm.eRepresentative pictures showing differences between isolated symbiosomes from WT andbid1. Symbiosomes were isolated from nodules inc. Bar=10 μm.fbid1symbiosomes were much shorter in length in the quantification assay of symbiosomes frome. Piano plot to show the minimum, 25th percentile, median, 75th percentile and maximum symbiosome lengths. Numbers of symbiosome analyzed were indicated respectively. “***”,P< 0.0001 in one-way ANOVA assay.gnifH::GUSreporter was not activated inbid1nodule cells. GUS staining was performed on WT andbid1nodules 21 days after inoculation withS. melilotiRM1021nifH::GUSat 21 dpi. Bar=750 μm.h, Expression ofNCR001was totally blocked inbid1nodule cells. qRT-PCR assay was performed using samples from nodules 21 dpi with ABS7hemA::LacZ. ND, not detected.iandj,Rhizobium ExoYandCtrAgenes were highly expressed inbid1nodule cells compared with WT. qRT-PCR assays were done using the same samples as inh. Forh,iandj, “**” and “***” meantP< 0.01 andP< 0.001 in Student’st-test, respectively. Data were represented as means ± SEM of three independent amplifications. Experiments were repeated at least 3 times with similar results. 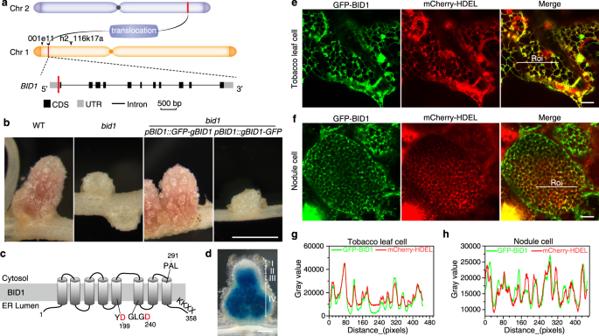Fig. 2:BID1encodes a nodule-specific, ER membrane-localized SPP. aA diagram showingBID1gene structure and the position of the target mutation in rough mapping.BID1was mapped to the upper arm of Chromosome 1, in the interval between markers 001e_01 and h2_116k17a. A 8,857-bp fragment from Chromosome 2, 44,572,929-44,581,777 bp, is inserted into the 5’ UTR ofMtrunA17_Chr1g0147151, 102 bp ahead of the start codon.bExpressingGFP-fused candidate gene genomic sequence driven by its own promoter could complement thebid1phenotype. Please note that GFP tag need be inserted at N-terminus of BID1. Bar=2 mm.cBID1 is a multi-transmembrane domain-containing SPP protein. The transmembrane domains were shown, and two conserved aspartate residues critical for peptidase activity were labeled red. PAL, a conserved motif important for peptidase activity; KKXX, the C-terminal ER membrane localization signal. Numbers indicated positions of the amino acids.dBID1is expressed exclusively in nodules in promoter-GUS reporter assay. Zone I, nodule meristem, Zone II, infection zone, the zone rhizobia infect nodule cells, Zone III, differentiation zone, the zone where symbiosomes undergo differentiation, Zone IV, fixation zone, the zone symbiosomes fix nitrogen. Bar=500 μm.eBID1 localized specifically at ER membrane when expressed in the leaves ofNicotiana benthamiana.N. benthamianaleaves co-transformed with35S::GFP-BID1andmCherry-HDELER reporter were analyzed under confocal microscopy at 2 days post-transformation. Bar=10 μm.f, BID1 localized to the ER membrane in nodule cells. A construct expressingpBID1::GFP-BID1together withmCherry-HDELreporter was transformed intobid1mutants. Bar=10 μm.gandhFluorescent intensity measurement of GFP-BID1 and mCherry-HDEL in indicated regions of tobacco leaf and nodule cells respectively. Fluorescent peaks of GFP-BID1 overlapped with mCherry-HDEL signals in both cell types. Fluorescent intensity was measured as grey value of pixels using ImageJ software. Roi, region of interest. Experiments were repeated more than 3 times with similar results. All the constructs used in this study were listed in Supplemental Table 1 , primers used for molecular cloning were listed in Supplemental Table 2 . Nodule sectioning, toluidine blue staining, X-gal and X-Gluc staining To section and stain the nodules, freshly picked nodules were vacuumed for 1 hour and fixed with 0.05 M nitrate phosphate buffer, pH 7.2, which contains 4% (w/v) paraformaldehyde and 5% (v/v) glutaraldehyde, for 12 hours at 4 °C. Fixed nodules were then dehydrated in the ethanol/dimethylbenzene solution series, and were embedded in paraffin subsequently. Then the samples were sliced into 5 μm thick sections on the Biosystems RM2245 microtome (Leica, Germany). Postsectioning, nodule slides were stained in 0.05% toluidine blue solution for 20 mins, and washed thoroughly in ddH 2 O. Stained nodule slides were checked and pictured using 3D Histech Pannoramic MIDI Slide Scanner (3DHISTECH, Hungary) following manufacturer’s instructions. X-Gal and X-Gluc staining were performed as previously described [50] , briefly fresh nodules were cut in half and stained with 0.8 mg/mL X-gal in Z′ buffer, or GUS staining buffer containing 10 mM/L X-Gluc respectively, for 12 hours at 37 °C. Samples were then washed with 100% ethanol until at least the roots were clear. The stained samples were analyzed and pictured, on the TL500 microsystem (Leica, Germany) equipped with a DMC6200 digital camera. Confocal microscopy analysis For confocal microscopy, nodules were hand-sectioned in half, the products were sectioned again for the observations. To determine symbiosome phenotypes through SYTO9 and PI staining, the sectioned nodules were stained with 10 mM/L SYTO9 and 5 mM/L PI for 5 mins. The excitation/emission wavelengths for SYTO9 and PI were set at 483 nm/503 nm and 493 nm/636 nm, respectively. For GFP and mCherry fluorescence, the excitation/emission wavelengths were 488 nm/507 nm and 587 nm/610 nm, respectively. For ER-Tracker Red staining (Beyotime, China), nodule samples were stained for 15 mins in the staining solution, the excitation and emission wavelengths were 587 nm and 615 nm, respectively. Samples were observed under a Ti-E + A1 MP Confocal Laser Scanning Microscope (Nikon, Japan). Quantitative Real-time PCR Quantitative Real-time (qRT) PCR was performed as previously described [51] , in brief total nodule RNA was extracted using TRIzol (Life Technology, the United States). Extracted RNA were treated with Turbo DNA-free kit (Invitrogen, the United States) to eliminate genomic DNA contamination. iScript cDNA synthesis kit (Bio-Rad, the United States) were used to synthesize the cDNA. All of the above procedures were done following manufacturers’ instructions. cDNA were diluted to a concentration of 0.5 μg/μL prior to PCR. qRT-PCR experiments were performed at a volume of 20 μL/reaction with 1 μg cDNA template. Experiments were performed using PerfectStart® Green qPCR SuperMix (Transgen, #AQ601-01) running on a Mastercycler EP Realplex system (Eppendorf, Germany). To rule out any non-specific amplifications, melting curves of PCR products were determined. Results were represented as means of threshold cycle values of three replicates. Relative expression of Medicago genes was normalized to PDF2 (MtrunA17_Chr6g0484701), for rhizobial genes, 16 S rRNA was used as the internal control. Primers used for qRT-PCR were listed in Supplemental Table 2 . Symbiosome protein extraction and proteomics assay Extraction of symbiosome proteins were performed as previously described [52] . In brief, freshly collected nodules were put into the pre-cooled (4 °C) extract solution I containing 0.5 M sucrose, 10 mM DTT, 50 mM Tris-HCl (pH 7.4), and 1% (v/v) protease inhibitor cocktail (P8340, Sigma-Aldrich), and were grounded thoroughly. Then samples were filtered through 2 layers of Microcloth (Calbiochem, the United States). Part of the filtered samples were centrifuged at 14,000 rpm for 20 mins and the supernatant was designated as total nodule proteins. For cytosol proteins, samples postfiltering were centrifuged at 10,000 g for 1 min, the supernatant was collected and labeled cytosol proteins. Then the pellets above centrifuge were re-suspended in a new solution with 1.5 M sucrose, 10 mM DTT, 50 mM Tris-HCl (pH 7.4) and 1% protease inhibitor cocktail (v/v), and centrifuged at 10,000 g for 90 seconds. 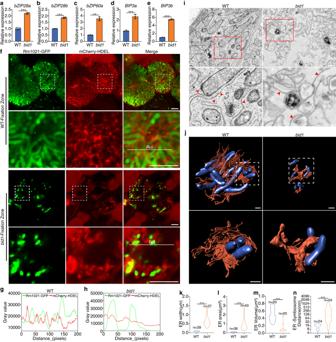Fig. 3: BID1 is required for proper ER-symbiosome proximal association. a-eIn qRT-PCR assay a group of ER stress-related marker genes were induced in 21 dpibid1nodules inoculated with ABS7hemA::LacZ. Error bars represent standard deviation from three biological replicates. “**” and “***”,P< 0.01 andP< 0.001 in Student’st-test respectively. Data were represented as means ± SEM of three independent amplifications.fConfocal microscopy analysis of ER structures in WT andbid1nodule cells. 14 dpi Rm1021pHC60-GFPinoculated mCherry-HDEL-expressing WT andbid1nodules were analyzed. For both panels, bar=10 μm. Roi, region of interest.gandhFluorescent intensity of symbiosome GFP and ER mCherry signals of indicated regions in WT andbid1respectively. Fluorescent intensity (grey value of pixels) was measured by ImageJ.iTEM assay results of ER and symbiosome structures in 14 dpi ABS7hemA::LacZ-inoculated WT andbid1nodule cells. For both panels, bar=1 μm.jReconstructed 3D structures of symbiosomes and ER in WT andbid1cells varied significantly. Overview of several ER and symbiosomes and zoomed-in structures of individual symbiosome and ER were shown. Symbiosomes were labelled in blue, ER in orange red. Structures were obtained through 3D reconstruction of AutoCUTS-SEM tomography data using Imaris software. Scal bar, 1 μm.kandlPiano charts showing differences in ER width and area between WT andbid1, respectively. ER width and area iniwere measured using ImageJ. “***”,P< 0.001 in One-way ANOVA assay.mMeasurement of ER volumes in WT andbid1by Imaris. “*”,P< 0.05 in one-way ANOVA assay. Numbers of ER analyzed were indicated.nAverage distance between ER membrane and symbiosome was much larger inbid1. ER-symbiosome distances were measured using Imaris. y-axis, logarithmic scores of ER-symbiosome distance to the base 2. “***”,P< 0.001 in one-way ANOVA assay. Fork,landn, numbers of ER analyzed were indicated. Form, 3D ER structures were evenly divided into 20 segments, volumes of each segment were determined. Experiments were repeated 3 times with similar results. The new pellets were re-suspended in extract solution I and labeled symbiosome proteins. 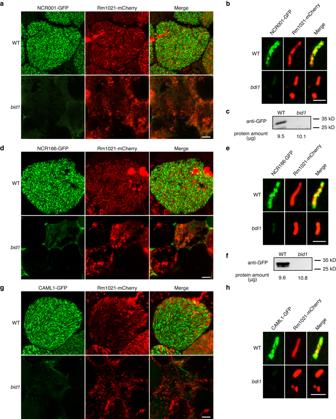Fig. 4: BID1 is required for the secretion pathway in nodule cells. a,dandgSecretion of NCR001, NCR166 and CAML1 were blocked inbid1nodule cells.GFP-fusedNCR001,NCR166andCAML1were expressed under theBID1promoter in WT andbid1, respectively. 14-day-old nodules inoculated withS. melilotiRm1021 mCherry were analyzed by confocal microscopy. Bar=10 μm.b,eandhGFP-fused NCR001, NCR166 and CAML1 could not be detected inbid1symbiosome. Symbiosomes were isolated from nodules ina,c, anderespectively, and analyzed by confocal microscopy. Bar=5 μm.candf, In Western blot assay of isolated symbiosome, secretion of NCR001 and NCR166 were blocked inbid1nodule cells.GFP-fusedNCR001,NCR166were expressed underBID1promoter in WT andbid1. Symbiosomes were isolated from 14-day-old nodules inoculated with ABS7hemA::LacZ. Protein samples were subjected to Western blot. Protein amounts loaded in each sample were labeled. Experiments were repeated more than 3 times with similar results. 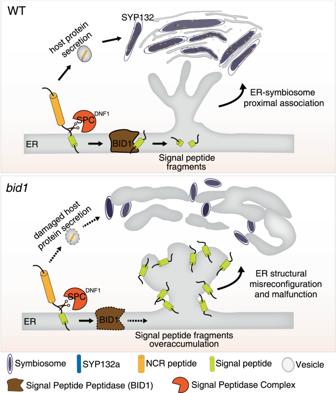Fig. 5: Diagram to summarize the function of BID1 in nodule cell ER reconfiguration and protein secretion. Nodule cells secrete a large number of proteins, e.g., NCR peptides, to symbiosomes to promote their differentiation. SP sequences could be found at the N terminus of these host proteins. The DNF1 nodule-specific SPC cleaves SP fragments from nascent sequences of host proteins to ensure proper folding and SYP132-mediated target protein secretion. On the ER membrane, remnant SP fragments will be cleaved by BID1, the nodule-specific SPP. In WT cells containing symbiosomes, ER forms an extensive web-like structure, closely surrounding differentiated symbiosomes. Inbid1mutant, with the nodule-specific SPP missed, ER structural reconfiguration and ER-symbiosomes proximal association are damaged, resulting in blockage of host protein secretion. In summary the nodule-specific SPP on ER membrane is critical for ER structural reconfiguration, ER-symbiosome proximal association, and host protein secretion. The concentration of protein samples were determined by Pierce™ BCA Protein Assay Kit according to manufacturers’ instructions. Equal amount of protein samples were boiled in 4× Laemmli buffer and were separated on SDS-PAGE gels. Proteins were then transferred to nitrocellulose membranes (Adventec) for immunoblotting analysis. The membrane was incubated with anti-GFP primary antibody (1:2000, GFP-Tag(7G9) mAb, Abmart) and secondary antibody (1:2500, Goat Anti-Mouse IgG HRP, Abmart), respectively and signals were visualized by enhanced chemiluminescence (Thermo Scientific) on an integrated chemiluminescent gel imaging system (OI600 Touch, Bio-OI). AutoCUTS-SEM sample preparation, serial sectioning, microscopy and 3D reconstruction 14 dpi WT and bid1 nodules inoculated with ABS hemA::LacZ were fixed 0.1 M Phosphate Buffer (pH 7.4) with 2.5% glutaraldehyde (v/v) and 2% paraformaldehydewith (v/v), and washed twice in Phosphate Buffer and ddH 2 O respectively. Fixed nodules were immersed in 1% OsO 4 (w/v) and 1.5% K 3 Fe(CN) 6 (w/v) aqueous solution at 4°C for 1 h, washed, incubated in filtered 1% thiocarbohydrazide aqueous solution (Sigma-Aldrich) at 25°C for 30 min, 1% unbuffered OsO 4 aqueous solution at 4°C for 1 h, and 1% UA aqueous solution at 25°C for 2 h. Then nodules were dehydrated with alcohol solution series (30, 50, 70, 80, 90, 100%, 100%), and pure acetone (twice), 10 min each at 4°C, infiltrated in graded mixtures (8:1, 5:1, 3:1, 1:1, 1:3, 1:5) of acetone and SPI-PON812 resin (21 mL SPI-PON812, 13 mL DDSA, 11 mL NMA, 1.5% BDMA), finally pure resin. Next nodules were embedded in pure resin (21 mL SPI-PON812, 13 mL DDSA, 10 mL NMA, 1.5% BDMA) and polymerized for 12 h at 45 °C, followed by 48 h at 60 °C. For 3D ultrastructure study, sections (449 for WT, 354 for bid1 , respectively) with thickness at 50 nm were prepared using ultramicrotome (UC7, Leica, Germany) with the AutoCUTS device (Zhenjiang Lehua Technology, China). Serial sections were automatically acquired by Helios Nanolab 600i dual-beam SEM (Thermo Fisher, the United States) with AutoSEE as the imaging software. Image parameters were set as follows, accelerating voltage 2 kV, beam current 0.69 nA, CBS detector, pixel size 6.7 nm for A17, 5.4 nm for bid1 , dwell time 3 microseconds. Alignment of serial sections was done by the registration function of MiRA-Align, all datasets were analyzed by Imaris software (Version 9.2.1). Statistics and reproducibility All quantitative data were presented as Mean ± S.D. The P values were calculated by Student’s t-test (unpaired and two-tailed) assays using GraphPad Prism 8 and the Excel software. A P value lower than 0.05 was considered statistically significant. “*” indicated P <  0.05, “**”, P <  0.01, “***”, P <  0.001, “****”, P <  0.0001, respectively. All experiments were replicated at least three times, representative data from the independent experiments were shown. No specific randomization or blinding protocols were used. Reporting summary Further information on research design is available in the Nature Portfolio Reporting Summary linked to this article.